Soluble amyloid precursor protein-α modulates β-secretase activity and amyloid-β generation In sporadic age-related forms of Alzheimer's disease (AD), it is unclear why amyloid-β (Aβ) peptides accumulate. Here we show that soluble amyloid precursor protein-α (sAPP-α) decreases Aβ generation by directly associating with β-site APP-converting enzyme (BACE)1, thereby modulating APP processing. Whereas specifically targeting sAPP-α using antibodies enhances Aβ production; in transgenic mice with AD-like pathology, sAPP-α overexpression decreases β-amyloid plaques and soluble Aβ. In support, immunoneutralization of sAPP-α increases APP amyloidogenic processing in these mice. Given our current findings, and because a number of risk factors for sporadic AD serve to lower levels of sAPP-α in brains of AD patients, inadequate sAPP-α levels may be sufficient to polarize APP processing towards the amyloidogenic, Aβ-producing route. Therefore, restoration of sAPP-α or enhancement of its association with BACE may be viable strategies to ameliorate imbalances in APP processing that can lead to AD pathogenesis. Alzheimer's disease (AD) affects 30 million worldwide with 5 million individuals in the United States alone (2011) and is characterized by pathologic hallmarks including β-amyloid plaques composed primarily of amyloid-β (Aβ) proteins as well as neurofibrillary tangles formed by abnormal phosphorylated tau proteins [1] , [2] . Aβ is thought to accumulate in toxic forms and damage neurons leading to synaptic dysfunction and neurodegeneration. Widespread neuronal loss ensues resulting in severe dementia and death. Much evidence implicates generation of Aβ as a critical component of AD pathogenesis [2] , [3] , [4] . Most inherited early-onset familial forms of AD result from autosomal dominant mutations in amyloid precursor protein (APP) or presenilin genes leading to a final common pathway involving excess Aβ accumulation [2] . Similarly, in sporadic age-related AD, risk factors for AD development, including metabolic dysfunction, cardiovascular disease and brain injury, also appear to favour Aβ accumulation and progressive neurodegeneration [5] , [6] , [7] , [8] , [9] , [10] . Aβ itself is produced by an alternative pathway whereby APP is cleaved first by β-site APP-converting enzyme (BACE) [11] . This process generates a carboxy (C)-terminal APP fragment (C99; β-CTF) and a large secreted amino (N)-terminal soluble fragment called sAPP-β. β-CTF is further processed by the γ-secretase complex, composed of presenilin, Aph-1, Nicastrin and Pen-2 proteins [12] , generating APP intracellular domain (AICD) and Aβ peptides of various lengths; of which Aβ 40 and Aβ 42 are believed to be predominant neurotoxic species in AD brains [13] . Under physiological conditions, Aβ is constitutively generated at relatively low levels. Hence, the majority of APP is processed by the non-amyloidogenic pathway. Here, α-secretase cleavage is performed by members of the ADAM metallopeptidase domain (ADAM) family yielding the α-secretase-generated C-terminal APP fragment (C83; α-CTF) and N-terminal portion of APP (soluble APP-α; sAPP-α) [14] . As α-secretase cuts APP within the Aβ region, Aβ generation is precluded. Subsequently, α-CTF is further processed by the γ-secretase complex to generate AICD and p3 peptides. Found to have neurotrophic and neuroprotective properties [15] , as well as the ability to enhance long-term potentiation [16] , sAPP-α is largely considered to have significant therapeutic potential [17] . Whereas in most familial forms of AD, where APP is 'genetically hijacked' by the amyloidogenic pathway, in sporadic age-related forms of the disease, it is unclear why Aβ accumulates. Previous investigations in sporadic age-related AD point to a number of AD risk factors, including combinations of oxidative stress, abnormal lipid metabolism, abnormal glucose metabolism, physical inactivity and cerebral hypoperfusion, all of which are also associated with suppressed sAPP-α [18] , [19] , [20] , [21] , [22] , [23] , [24] , [25] , [26] , [27] , [28] , [29] , [30] . Furthermore, α-secretase mutations have been associated with familial late-onset AD [31] . These data, in combination with previous data implying that sAPP-α has a role in the autoregulation of APP processing [32] , [33] , [34] , motivated our current investigation to determine how sAPP-α regulates APP processing. Here, we investigated the effects of sAPP-α treatment on APP processing in Chinese hamster ovary (CHO) cells overexpressing wild-type APP (APP wt ) or Swedish mutant APP (APP swe ), with or without, human wild-type PS1 (PS1 wt ) or mutant PS1 (PS1 mut ). We found that purified human recombinant sAPP-α (hsAPP-α) decreases Aβ and β-CTF production, implicating β-secretase modulation. In support, immunoprecipitation (IP) analysis revealed that sAPP-α directly interacts with BACE1 and interferes with the BACE1/APP interaction, resulting in decreased Aβ and β-CTF production. Moreover, in aged transgenic mice overexpressing APP swe and PS1 mut (PSAPP mice), elevated central nervous system (CNS) sAPP-α mitigated β-amyloid pathology. In contrast, a specific antibody targeting sAPP-α was sufficient to drive amyloidogenic APP processing in PSAPP mice. In sum, these data suggest that inadequate levels of sAPP-α leave this model more vulnerable to AD-like pathology. This has strong clinical implications as many known AD risk factors, including oxidative stress, abnormal lipid metabolism, abnormal glucose metabolism, physical inactivity and cerebral hypoperfusion, are also associated with suppressed sAPP-α levels [18] , [19] , [20] , [21] , [22] , [23] , [24] , [25] , [26] , [27] , [28] , [29] , [30] . sAPP-α decreases Aβ species and β-CTF in vitro A product of non-amyloidogenic APP processing, sAPP-α, exerts both neuroprotective and neurotrophic properties [14] , [15] , [34] , [35] , [36] , [37] , [38] , [39] . Owing to these properties, evidence for several mechanisms appear to be determinative, yet of particularly intrigue is evidence implicating sAPP-α itself in modulation of the parent APP molecule [32] , [33] , [34] . Thus, we endeavoured to test whether sAPP-α could affect Aβ generation. To address this question, we first employed purified human recombinant sAPP-α (hsAPP-α) [15] , [35] , [40] , [41] produced in the human embryonic kidney (HEK) cell line 293. CHO cells stably overexpressing both Swedish mutant APP and wild-type human PS1 (CHO/APP swe /PS1 wt ) were treated with a dose range (0–2 nM) of hsAPP-α for 4 h followed by examination of APP metabolites. Immunoblot (IB) analysis showed that treatment with hsAPP-α mitigates generation of both Aβ 40 and Aβ 42 ( Fig. 1a ). Heat-inactivated hsAPP-α did not affect Aβ generation. We confirmed these findings with sandwich ELISA ( Fig. 1b ), which showed dramatic reductions in both Aβ 40 and Aβ 42 levels in cells treated with hsAPP-α compared with heat-inactivated hsAPP-α. Next, in an effort to determine whether hsAPP-α could affect β-, γ- or α-secretase APP cleavage events, we monitored APP C-terminal fragments (CTFs) by IB analysis ( Fig. 1c ). Densitometry analysis of these data showed that hsAPP-α dramatically decreases β-CTF generation compared with controls ( Fig. 1d ). 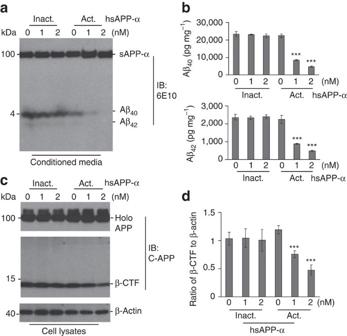Figure 1: sAPP-α inhibits β-secretase cleavage of APPin vitro. CHO cells expressing APPsweand wild-type human PS1 (CHO/APPswe/PS1wt) cells were treated with active (act.) or inactive (inact.) hsAPP-α recombinant protein at 0, 1 and 2 nM as indicated for 4 h. Secreted Aβ40, 42peptides in the cell culture medium were analysed by (a) IB and (b) Aβ ELISA analyses. The Aβ ELISA results are represented as the mean±s.d. of picograms of Aβ40or Aβ42per milligram of total intracellular protein after hsAPP-α protein treatment. In addition, these results are representative of four independent experiments withn=3 for each condition. (c) Cell lysates were prepared and APP CTFs were analysed by IB using a rabbit polyclonal antibody against C-terminal APP (pAb751/770, C-APP). This β-CTF band was further confirmed by the additional IB using 6E10 antibody. (d) Relative ratio (mean±s.d.) of β-CTF to β-actin was calculated by densitometry analysis. The results are representative of three independent experiments withn=3 for each condition. One-way analysis of variance followed bypost hoccomparison revealed significant differences between 1 or 2 and 0 nM hsAPP-α protein treatment in both of Aβ40, 42reduction and relative ratio of β-CTF to β-actin (***P<0.001, full-length APP, holo APP). Figure 1: sAPP-α inhibits β-secretase cleavage of APP in vitro . CHO cells expressing APP swe and wild-type human PS1 (CHO/APP swe /PS1 wt ) cells were treated with active (act.) or inactive (inact.) hsAPP-α recombinant protein at 0, 1 and 2 nM as indicated for 4 h. Secreted Aβ 40, 42 peptides in the cell culture medium were analysed by ( a ) IB and ( b ) Aβ ELISA analyses. The Aβ ELISA results are represented as the mean±s.d. of picograms of Aβ 40 or Aβ 42 per milligram of total intracellular protein after hsAPP-α protein treatment. In addition, these results are representative of four independent experiments with n =3 for each condition. ( c ) Cell lysates were prepared and APP CTFs were analysed by IB using a rabbit polyclonal antibody against C-terminal APP (pAb751/770, C-APP). This β-CTF band was further confirmed by the additional IB using 6E10 antibody. ( d ) Relative ratio (mean±s.d.) of β-CTF to β-actin was calculated by densitometry analysis. The results are representative of three independent experiments with n =3 for each condition. One-way analysis of variance followed by post hoc comparison revealed significant differences between 1 or 2 and 0 nM hsAPP-α protein treatment in both of Aβ 40, 42 reduction and relative ratio of β-CTF to β-actin (*** P <0.001, full-length APP, holo APP). Full size image Targeting sAPP-α enhances Aβ generation Considering our observations that hsAPP-α treatment decreases Aβ species and APP β-CTF generation, previous investigations identifying mutations in sAPP-α-generating enzyme ADAM10 in familial late-onset AD [31] , and evidence suggesting that a number of risk factors for sporadic forms of AD may serve to lower levels of sAPP-α in brains of AD patients [18] , [19] , [20] , [21] , [22] , [23] , [24] , [25] , [26] , [27] , [28] , [29] , [30] , we hypothesized that the loss of sAPP-α would be sufficient to drive amyloidogenic APP processing. To test this hypothesis, before treatment of CHO cells expressing wild-type APP (CHO/APP wt cells), we first immunodepleted hsAPP-α protein with an antibody specifically against C-terminus of sAPP-α (2B3 antibody), or isotype-matched IgG 2b control antibody, utilizing Protein-G Sepharose beads. After treatment, the conditioned media and cell lysates were prepared and assayed for APP metabolites. An increase in Aβ 40 and Aβ 42 was only observed in the cells receiving hsAPP-α preparations immunodepleted with 2B3 antibody, but not in those immunodepleted with isotype-matched IgG 2b control antibody ( Fig. 2a and b ). In accordance with these findings, APP β-CTF was only increased in the cells treated with hsAPP-α immunodepleted with 2B3 antibody, but not in the cells treated with IgG 2b immunodepleted hsAPP-α ( Fig. 2c and d ). These results indicated that immunodepletion of hsAPP-α using 2B3 antibody attenuates the anti-amyloidogenic effect of hsAPP-α on APP processing. As a confirmation, we have replicated this result in CHO/APP swe /PS1 wt cells utilizing an antibody against Aβ 1−17 peptide (6E10 antibody) ( Supplementary Fig. S1 ). 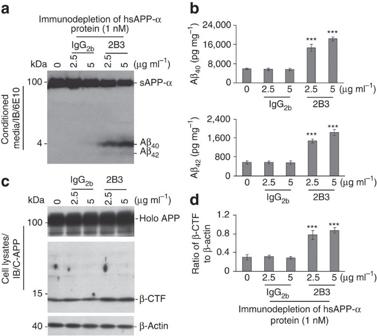Figure 2: Immunodepleted sAPP-α attenuates sAPP-α effects on APP modulationin vitro. Active hsAPP-α protein at 1 nM was incubated with an anti-C-terminal sAPP-α-specific 2B3 antibody or isotype-matched IgG2bcontrol antibody at 0, 2.5 and 5 μg ml−1at 37 C for 30 min. The protein-G sepharose beads were used to pull-down sAPP-α antibody and isotype-matched IgG2bcontrol, as well as their associated proteins. This was followed by high-speed centrifugation at 15,000gfor 10 min, and the supernatants were collected and determined to be IgG antibody-free by IB analysis using an antibody against IgG2b. These supernatants were used to treat CHO cells expressing human wild-type APP (CHO/APPwt) for 12 h. Cell-cultured supernatants were collected and subjected to (a) Aβ IB analysis using 6E10 antibody and (b) the Aβ ELISA results are represented as the mean±s.d. of picograms of Aβ40or Aβ42per milligram of total intracellular protein after the 2B3- or control IgG2b-immunodepleted hsAPP-α protein treatment. (c) Cell lysates were prepared and APP CTFs were analysed by IB using pAb751/770 (C-APP). (d) Relative ratio (mean±s.d.) of β-CTF to β-actin was calculated by densitometry analysis. Forbandd, the results as presented are representative of two independent experiments withn=3 for each condition. One-way analysis of variance followed bypost hoccomparison revealed significant differences between 2B3-immunodepleted hsAPP-α protein treatment at either 2.5 or 5 μg ml−1and control IgG2b-immunodepleted hsAPP-α protein as measured by either Aβ levels or ratio of β-CTF to β-actin (***P<0.001, full-length APP, holo APP). Figure 2: Immunodepleted sAPP-α attenuates sAPP-α effects on APP modulation in vitro. Active hsAPP-α protein at 1 nM was incubated with an anti-C-terminal sAPP-α-specific 2B3 antibody or isotype-matched IgG 2b control antibody at 0, 2.5 and 5 μg ml −1 at 37 C for 30 min. The protein-G sepharose beads were used to pull-down sAPP-α antibody and isotype-matched IgG 2b control, as well as their associated proteins. This was followed by high-speed centrifugation at 15,000 g for 10 min, and the supernatants were collected and determined to be IgG antibody-free by IB analysis using an antibody against IgG 2b . These supernatants were used to treat CHO cells expressing human wild-type APP (CHO/APP wt ) for 12 h. Cell-cultured supernatants were collected and subjected to ( a ) Aβ IB analysis using 6E10 antibody and ( b ) the Aβ ELISA results are represented as the mean±s.d. of picograms of Aβ 40 or Aβ 42 per milligram of total intracellular protein after the 2B3- or control IgG 2b -immunodepleted hsAPP-α protein treatment. ( c ) Cell lysates were prepared and APP CTFs were analysed by IB using pAb751/770 (C-APP). ( d ) Relative ratio (mean±s.d.) of β-CTF to β-actin was calculated by densitometry analysis. For b and d , the results as presented are representative of two independent experiments with n =3 for each condition. One-way analysis of variance followed by post hoc comparison revealed significant differences between 2B3-immunodepleted hsAPP-α protein treatment at either 2.5 or 5 μg ml −1 and control IgG 2b -immunodepleted hsAPP-α protein as measured by either Aβ levels or ratio of β-CTF to β-actin (*** P <0.001, full-length APP, holo APP). Full size image To further test our hypothesis that the loss of sAPP-α is sufficient to drive amyloidogenic APP processing, we next sought the immunoneutralization of endogenously produced sAPP-α. Separate groups of CHO/APP wt cells were treated directly with either a sAPP-α-specific 2B3 antibody or isotype-matched IgG 2b control antibody for 12 h. Aβ release into supernatants from these cells was analysed by IB analysis ( Fig. 3a and b ). This analysis indicated that immunoneutralization of endogenous sAPP-α activity increases the generation of Aβ. Analysis of cell lysates showed that immunoneutralization of endogenous sAPP-α significantly enhances APP β-CTF generation ( Fig. 3c ) and β-CTF/β-actin ratios ( Fig. 3d ) compared with cells treated with isotype-matched IgG 2b control antibody. In addition, we have repeated this experiment in CHO/APP swe /PS1 wt cells utilizing 6E10 antibody ( Supplementary Fig. S2 ). Altogether, these data show that immunoneutralization of endogenous sAPP-α activity is sufficient to drive amyloidogenic APP processing. 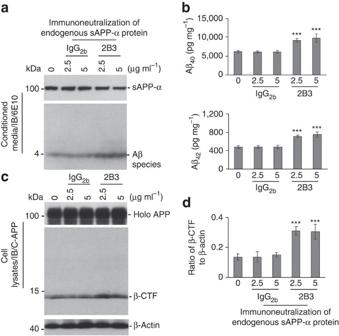Figure 3: Immunoneutralization of endogenous sAPP-α promotes APP amyloidogenic processing. CHO/APPwtcells were treated with 2B3 or isotype-matched IgG2bcontrol antibody for 12 h as indicated. (a) Aβ species were analysed in conditioned media from the treated CHO/APPwtcells by IB analysis using 6E10 antibody. (b) The Aβ ELISA results are represented as the mean±s.d. of picograms of Aβ40or Aβ42per milligram of total intracellular protein after the 2B3 antibody treatment. In addition, these results are representative of three independent experiments withn=3 for each condition. (c) Cell lysates were prepared and APP CTFs were analysed by IB analysis using pAb751/770 (C-APP). (d) Densitometry shows the ratio (mean±s.d.) of β-CTF to β-actin. Forbandd, the results as presented are representative of three independent experiments withn=3 for each condition. One-way analysis of variance followed bypost hoccomparison revealed a significant difference between the 2B3 antibody at either 2.5 or 5 μg ml−1and isotype-matched IgG2bcontrol antibody treatment conditions (***P<0.001, full-length APP, holo APP). Figure 3: Immunoneutralization of endogenous sAPP-α promotes APP amyloidogenic processing. CHO/APP wt cells were treated with 2B3 or isotype-matched IgG 2b control antibody for 12 h as indicated. ( a ) Aβ species were analysed in conditioned media from the treated CHO/APP wt cells by IB analysis using 6E10 antibody. ( b ) The Aβ ELISA results are represented as the mean±s.d. of picograms of Aβ 40 or Aβ 42 per milligram of total intracellular protein after the 2B3 antibody treatment. In addition, these results are representative of three independent experiments with n =3 for each condition. ( c ) Cell lysates were prepared and APP CTFs were analysed by IB analysis using pAb751/770 (C-APP). ( d ) Densitometry shows the ratio (mean±s.d.) of β-CTF to β-actin. For b and d , the results as presented are representative of three independent experiments with n =3 for each condition. One-way analysis of variance followed by post hoc comparison revealed a significant difference between the 2B3 antibody at either 2.5 or 5 μg ml −1 and isotype-matched IgG 2b control antibody treatment conditions (*** P <0.001, full-length APP, holo APP). Full size image sAPP-α interacts and inhibits BACE1 We next aimed to investigate the mechanism by which sAPP-α suppressed Aβ generation. Given the observed decreased Aβ production without accumulation of β-CTF in response to sAPP-α ( Fig. 1 ), we hypothesized that sAPP-α could inhibit β-secretase activity in some manner, be it directly or indirectly [43] . BACE1 is a type I transmembrane aspartyl protease predominately responsible for processing APP into sAPP-β and β-CTF (C99) in the CNS. β-CTF is subsequently cleaved by the γ-secretase, releasing Aβ species of various lengths [11] . In light of recent findings indicating that a C-terminal BACE1 inhibition domain is contained within APP [44] , we reasoned that because sAPP-α, but not sAPP-β, also contains this domain, sAPP-α could directly or indirectly interact with BACE1 and decrease BACE1 activity. To investigate whether sAPP-α interacts with BACE1, we treated CHO/APP wt cells with hsAPP-α or heat-inactivated hsAPP-α protein and then collected cell lysates for analyses. As shown in Fig. 4a , cell lysates subjected to IP for BACE1 followed by IB for sAPP-α displayed strong coprecipitation of sAPP-α. Accordingly, IP for sAPP-α followed by IB for BACE1 showed coprecipitation of BACE1 ( Fig. 4b ). However, these coprecipitions were markedly reduced in heat-inactivated hsAPP-α condition. 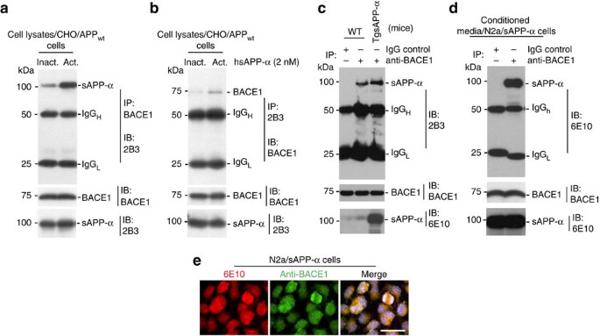Figure 4: sAPP-α interacts with BACE1 in cultured cells. CHO/APPwtcells were treated with active or inactive hsAPP-α protein at 2 nM for 8 h. The cell lysates were IP with either (a) anti-C-terminal BACE1 (BACE1) antibody or (b) 2B3 antibody and then probed with 2B3 or BACE1 antibody. These results as presented are representative of three independent experiments withn=3 for each condition. (c) Mouse brain homogenates prepared from TgsAPP-α mice and wild-type littermates (WT), and subjected to IP with BACE1 antibody or isotype control IgG for BACE1 followed by IB for sAPP-α using 2B3 antibody. The results as presented are representative of results obtained for three mice per group. (d) The conditioned media collected from cultured N2a/sAPP-α cells were subjected to IP with BACE1 antibody or isotype control IgG for BACE1 followed by IB with 6E10 antibody. As indicated below these blots, IB analyses demonstrate total protein levels of around 75 kDa BACE1 and 100 kDa sAPP-α in the different cell lysates, conditioned media or mouse brain homogenates. (e) sAPP-α strongly associates with BACE1 in N2a cell line stably transfected with human sAPP-α (N2a/sAPP-α cells). The cultured N2a/sAPP-α cells were fixed and imaged in independent channels using a confocal microscope equipped with Normarski optics. Merged images showed strong localization of both 6E10 antibody and BACE1 antibody-positive N2a/sAPP-α cells (scale bar: 50 μm). Figure 4: sAPP-α interacts with BACE1 in cultured cells. CHO/APP wt cells were treated with active or inactive hsAPP-α protein at 2 nM for 8 h. The cell lysates were IP with either ( a ) anti-C-terminal BACE1 (BACE1) antibody or ( b ) 2B3 antibody and then probed with 2B3 or BACE1 antibody. These results as presented are representative of three independent experiments with n =3 for each condition. ( c ) Mouse brain homogenates prepared from TgsAPP-α mice and wild-type littermates (WT), and subjected to IP with BACE1 antibody or isotype control IgG for BACE1 followed by IB for sAPP-α using 2B3 antibody. The results as presented are representative of results obtained for three mice per group. ( d ) The conditioned media collected from cultured N2a/sAPP-α cells were subjected to IP with BACE1 antibody or isotype control IgG for BACE1 followed by IB with 6E10 antibody. As indicated below these blots, IB analyses demonstrate total protein levels of around 75 kDa BACE1 and 100 kDa sAPP-α in the different cell lysates, conditioned media or mouse brain homogenates. ( e ) sAPP-α strongly associates with BACE1 in N2a cell line stably transfected with human sAPP-α (N2a/sAPP-α cells). The cultured N2a/sAPP-α cells were fixed and imaged in independent channels using a confocal microscope equipped with Normarski optics. Merged images showed strong localization of both 6E10 antibody and BACE1 antibody-positive N2a/sAPP-α cells (scale bar: 50 μm). Full size image In order to confirm a physiologically relevant BACE1 and sAPP-α interaction, we performed IP on brain homogenates from TgsAPP-α mice and wild-type littermates utilizing an anti-BACE1 antibody for BACE1 and then IB with an anti-C-terminal sAPP-α-specific 2B3 antibody for sAPP-α. The results displayed strong coprecipitation of sAPP-α in both TgsAPP-α mice and wild-type littermates ( Fig. 4c ). Finally, we generated a stable N2a cell line overexpressing hsAPP-α (N2a/sAPP-α). Cell supernatants collected from these cells were subjected to IP for BACE1 and then IB for sAPP-α. They displayed strong coprecipitation of sAPP-α compared with isotype IgG control ( Fig. 4d ). Moreover, we performed immunofluorescence staining on these cells and visualized both human sAPP-α and BACE1, and observed considerable colocalization of sAPP-α and BACE1 in these cells ( Fig. 4e ). These findings indicate that sAPP-α interferes with amyloidogenic APP processing through direct or indirect interaction with BACE1. In addition, this experiment was repeated in CHO/APP swe /PS1 wt cells. Again, a strong interaction of BACE1 with sAPP-α was further confirmed in both conditioned media ( Supplementary Fig. S3a ) and cell lysates ( Supplementary Fig. S3b ). We next wondered whether BACE1/APP interaction was affected by sAPP-α treatment. Remarkably, the cell lysates prepared from CHO/APP swe /PS1 wt cells that had been treated with sAPP-α, followed by IP for BACE1 and IB for C-terminal APP showed a dramatic reduction in coprecipitation of full-length APP, an effect not observed with heat-inactivated sAPP-α. Moreover, confirming our earlier CTF interpretation, decreased β-CTF correlated with high BACE1/sAPP-α- and low BACE1/APP-interacting conditions created by sAPP-α treatment ( Supplementary Fig. S3b ). These results further support our hypothesis that sAPP-α interacts and inhibits BACE1 activity in terms of APP processing. sAPP-α suppresses β-amyloid pathology in AD mice To determine whether sAPP-α reduces amyloidogenic APP processing in vivo , we generated transgenic mice overexpressing human sAPP-α (TgsAPP-α mice) in CNS tissues, and crossed them with the double transgenic APP swe /PSEN1 ΔE9 (PSAPP) AD mouse model. Female triple transgenic and littermate control mice were aged to 8 months, euthanized and AD-like pathology was characterized. Overexpression of sAPP-α substantially decreases cortical and hippocampal β-amyloid plaques, as well as Aβ oligomeric forms visualized by immunohistochemistry (4G8 and an anti-Aβ oligomer antibody OC), and reduces fibrillar Aβ species visualized by Thioflavin-S staining ( Fig. 5a–c ). Correspondingly, brain extracts prepared from these same mice were analysed for soluble and insoluble Aβ 40, 42 by ELISA ( Fig. 6a ) and IB utilizing 6E10 antibody ( Fig. 6b ). sAPP-α overexpression also significantly decreases Aβ 40 and Aβ 42 , both soluble and insoluble Aβ levels, compared with PSAPP littermate controls. In order to test whether sAPP-α suppresses BACE1-mediated APP processing in vivo , we further analysed APP CTF expression ( Fig. 6b ). Overexpression of sAPP-α results in dramatic inhibition of β-CTF. 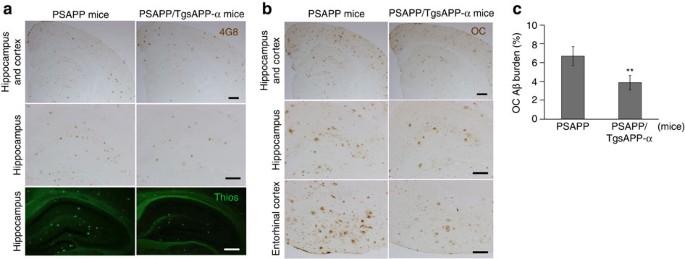Figure 5: sAPP-α reduces β-amyloid pathology in a mouse model of AD. (a) Mouse brain sections from PSAPP and PSAPP/TgsAPP-α mice were stained with anti-Aβ17−24antibody [4G8: brown, up (scale bar: 50 μm) and middle panels (scale bar: 50 μm)] or Thioflavin S [ThioS: green signal, bottom panel (scale bar: 50 μm)] at 8 months of age. (b) Mouse brain sections from PSAPP and PSAPP/TgsAPP-α mice were stained with Aβ OC antibody (brown signal). (c) Percentage of Aβ OC antibody immunoreactive plaques from hippocampus and cortex (mean±s.d.;n=5 females per group) was quantified by image analysis. At-testcfor independent samples revealed significances between groups (**P<0.01). Figure 5: sAPP-α reduces β-amyloid pathology in a mouse model of AD. ( a ) Mouse brain sections from PSAPP and PSAPP/TgsAPP-α mice were stained with anti-Aβ 17−24 antibody [4G8: brown, up (scale bar: 50 μm) and middle panels (scale bar: 50 μm)] or Thioflavin S [ThioS: green signal, bottom panel (scale bar: 50 μm)] at 8 months of age. ( b ) Mouse brain sections from PSAPP and PSAPP/TgsAPP-α mice were stained with Aβ OC antibody (brown signal). ( c ) Percentage of Aβ OC antibody immunoreactive plaques from hippocampus and cortex (mean±s.d. ; n =5 females per group) was quantified by image analysis. A t -test c for independent samples revealed significances between groups (** P <0.01). 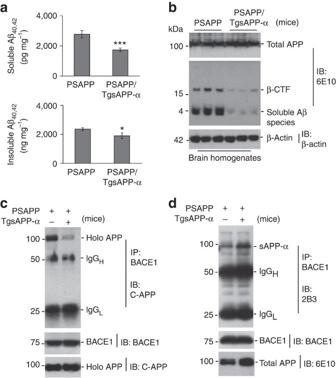Figure 6: sAPP-α inhibits amyloidogenic APP processingin vivo. Mouse brain homogenates were prepared from 8-month-old PSAPP and PSAPP/TgsAPP-α mice. (a) Total soluble and insoluble Aβ40, 42were biochemically assessed in brain homogenates by ELISA and (b) total soluble Aβ species from brain homogenates were analysed by IB using 6E10 antibody. For (a), data are presented as picograms (soluble Aβ40,42) or nanograms (insoluble Aβ40,42) per milligrams of protein (mean±s.d.;n=5 females per group). Mouse brain homogenates (200 μg) per mouse were IP with (c) an anti-C-terminal BACE1 antibody for BACE1, followed by IB analysis with pAb751/770 (C-APP) for full-length APP (holo APP) (d) with an anti-C-terminal BACE1 antibody for BACE1, followed by IB for sAPP-α with 2B3 antibody. As indicated below this figure, IB analyses demonstrate total protein levels of around 100 kDa total APP by 6E10 antibody and 75 kDa BACE1 in the different mouse brain homogenates. All results as presented are representative of results obtained for five mice per group (*P<0.05, ***P<0.001). Full size image Figure 6: sAPP-α inhibits amyloidogenic APP processing in vivo . Mouse brain homogenates were prepared from 8-month-old PSAPP and PSAPP/TgsAPP-α mice. ( a ) Total soluble and insoluble Aβ 40, 42 were biochemically assessed in brain homogenates by ELISA and ( b ) total soluble Aβ species from brain homogenates were analysed by IB using 6E10 antibody. For ( a ), data are presented as picograms (soluble Aβ 40,42 ) or nanograms (insoluble Aβ 40,42 ) per milligrams of protein (mean±s.d. ; n =5 females per group). Mouse brain homogenates (200 μg) per mouse were IP with ( c ) an anti-C-terminal BACE1 antibody for BACE1, followed by IB analysis with pAb751/770 (C-APP) for full-length APP (holo APP) ( d ) with an anti-C-terminal BACE1 antibody for BACE1, followed by IB for sAPP-α with 2B3 antibody. As indicated below this figure, IB analyses demonstrate total protein levels of around 100 kDa total APP by 6E10 antibody and 75 kDa BACE1 in the different mouse brain homogenates. All results as presented are representative of results obtained for five mice per group (* P <0.05, *** P <0.001). Full size image Finally, we determined whether sAPP-α could interfere with BACE1/APP association in vivo through analysis of these same brain extracts utilizing IP for BACE1 followed by IB for C-terminal APP. Here, our findings clearly indicate a dramatic reduction in coprecipitation of full-length (holo) APP with BACE1 in PSAPP/sAPP-α mice compared with PSAPP littermate controls ( Fig. 6c ). Most importantly, IB utilizing an anti-C-terminal sAPP-α-specific 2B3 antibody for sAPP-α reveals a significant increase in coprecipitation of sAPP-α with BACE1 in PSAPP/sAPP-α mice compared with PSAPP littermates. These data altogether indicate that sAPP-α interferes with amyloidogenic APP processing through association with BACE1 by preventing association and amyloidogenic proteolysis of APP ( Fig. 6d ). Immunoneutralization of sAPP-α enhances Aβ generation in vivo The above findings suggest that sAPP-α is able to decrease amyloidogenic APP processing in vivo . We hypothesized based on our in vitro and in vivo findings that the inverse was also true, specifically that loss of sAPP-α function could drive amyloidogenic APP processing. Consistent with this hypothesis, 8-month-old female PSAPP mice treated intracerebroventricular (i.c.v.) with a sAPP-α-specific 2B3 antibody for 48 h displayed enhanced amyloidogenic APP processing compared with control (isotype-matched IgG 2b control antibody). Specifically, immunoneutralization of sAPP-α increases soluble Aβ 40, 42 levels by IB analysis ( Fig. 7a and b ) compared with PSAPP mice receiving i.c.v. isotype-matched IgG 2b control antibody. In accordance with these findings, β-CTF generation was enhanced with sAPP-α immunoneutralization ( Fig. 7c ). In addition, our preliminary study also showed that PSAPP mice i.c.v. treated with 6E10 exhibit an increase in soluble Aβ and enhancement of β-CTF generation. Altogether, these data show that sAPP-α immunoneutralization enhances amyloidogenic APP processing. 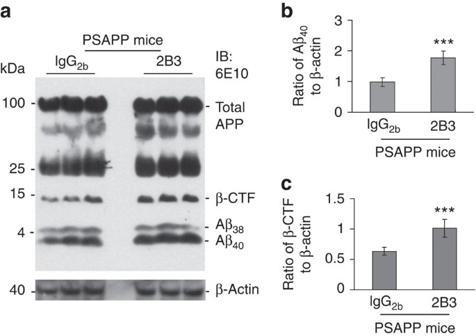Figure 7: Antibody targeting of sAPP-α promotes amyloidogenic APP processingin vivo. PSAPP mice (three female mice per group) at 8 months of age were i.c.v. injected with 2B3 antibody or isotype-matched IgG2bcontrol antibody at 5 μg ml−1and killed at 48 h after the injection. (a) Mouse brain homogenates were prepared from these mice and subjected to IB analysis for APP processing. IB using 6E10 antibody shows total APP and three bands corresponding to β-CTF and soluble Aβ species 38 and 40. Densitometry analysis shows the ratios of Aβ40to β-actin (b) and β-CTF to β-actin (c). At-test revealed significant differences in either ratio of Aβ40to β-actin or β-CTF to β-actin between 2B3 antibody- and control IgG2bantibody-i.c.v. injected PSAPP mice (***P<0.001). Figure 7: Antibody targeting of sAPP-α promotes amyloidogenic APP processing in vivo . PSAPP mice (three female mice per group) at 8 months of age were i.c.v. injected with 2B3 antibody or isotype-matched IgG 2b control antibody at 5 μg ml −1 and killed at 48 h after the injection. ( a ) Mouse brain homogenates were prepared from these mice and subjected to IB analysis for APP processing. IB using 6E10 antibody shows total APP and three bands corresponding to β-CTF and soluble Aβ species 38 and 40. Densitometry analysis shows the ratios of Aβ 40 to β-actin ( b ) and β-CTF to β-actin ( c ). A t -test revealed significant differences in either ratio of Aβ 40 to β-actin or β-CTF to β-actin between 2B3 antibody- and control IgG 2b antibody-i.c.v. injected PSAPP mice (*** P <0.001). Full size image Our findings suggest that sAPP-α can promote non-amyloidogenic APP processing. Our initial indication of this was evidenced in cells overexpressing APP swe and PS1 wt (CHO/APP swe /PS1 wt cells) where exogenous hsAPP-α inhibited Aβ 40, 42 and β-CTF production ( Fig. 1 ), a pattern indicative of suppression of β-secretase APP cleavage ( Fig. 1c and d ). Underlying this, we found a physical association between sAPP-α and BACE1 in vitro ( Fig. 4a, b and d ), and in both TgsAPP-α mice and wild-type littermates and at endogenous levels ( Fig. 4c ), suggesting a physiologically relevant phenomenon. Indeed, immunoprecipitaton (IP) with an anti-BACE1 antibody and IB with an anti-C-terminal sAPP-α-specific 2B3 antibody exhibited strong coprecipitation of sAPP-α in both TgsAPP-α mice and wild-type littermates ( Fig. 4c ). These results strongly support a physiologically relevant BACE1 and sAPP-α interaction at endogenous levels. Furthermore, others have already shown that APP itself contains a unique C-terminal sequence found to decrease BACE1 activity [44] lending further credence to our data and conclusions as this region is also present in sAPP-α but not in sAPP-β. In further support, BACE1 has been shown to be secreted in conditioned media [45] , [46] , [47] , [48] and thus binding of sAPP-α to BACE1 ( Fig. 4d and e ) could occur in either the extracellular compartment, at the membrane or presumably during endocytosis. Reduced interaction of BACE1 with full-length APP would be expected if sAPP-α could interfere with their association. Indeed, we found that PSAPP mice overexpressing sAPP-α show decreased BACE1 and full-length APP interaction ( Fig. 6c ), whereas PSAPP mice exhibited the opposite ( Fig. 6c and d ). Furthermore, suppression of sAPP-α function via antibody immunodepletion of exogenous ( Fig. 2 ), and immunoneutralization of endogenously generated sAPP-α ( Fig. 3 ) enhanced Aβ production. These findings demonstrate for the first time that sAPP-α may be involved in a positive feedback loop whereby it promotes its own production by inhibiting BACE1's ability to interact with and proteolyze full-length APP at physiological levels. To confirm this physiological relevance, we conducted the coprecipitation experiments both in conditioned media and brain homogenates. Specifically, we performed coprecipitation of CHO/APP wt cell lysates utilizing the specific sAPP-α antibody (2B3) that neither recognizes Aβ nor full-length APP. These coprecipitation data suggested that sAPP-α interacts with BACE1 in some manner in these cell culture systems and this interaction is associated with decreased Aβ generation. However, these data do not completely rule out the possibility that intermediate factors are required for inhibition of BACE1's association and proteolysis of APP. In light of the attenuation of sAPP-α's Aβ lowering effects by immunoneutralization utilizing 2B3 antibody ( Fig. 3 ), as well as similar findings with utilizing an antibody against Aβ 1−17 peptide (6E10 antibody) ( Supplementary Fig. S2 ), intermediate factors presumably still present in this immunoneutralization paradigm did not appear to mitigate the effects of directly targeting sAPP-α. The possibility of the immunodepletion antibody, 2B3, interfering with either Aβ generation or its measurement by ELISA exists, but at an extremely low likelihood given that we found no detectable IgG by IB ( Fig. 2 and Supplementary Fig. S1 ). In this regard, one may also speculate that contaminating sAPP-β may be present, which may be confounding our data. However, this is also likely not occurring because this peptide would not be removed through immunodepletion of sAPP-α with the specific 2B3 antibody and thus suppression of Aβ peptides should still be observed, yet the results support the opposite conclusion ( Fig. 2 and Supplementary Fig. S1 ). The possibility of another receptor, in addition or alternative to BACE1, being responsible for sAPP-α's Aβ lowering effects exists since APP and its metabolites are known to exhibit multimodal effects and multiple binding partners. Importantly, however, the immunoneutralization results using sAPP-α-specific antibody ( Fig. 3 ) suggested that no regions, other than the region at or near the target epitope at the C-terminal of sAPP-α, appear required for sAPP-α's anti-amyloidogenic effects. Further, the regions bound by the immunoneutralization antibodies are regions of sAPP-α characterized to have a unique BACE1 inhibition sequence [44] . In contrast, IgG 2b immunoneutralization or immunodepletion of endogenous or exogenous sAPP-α, respectively, yielded no changes in APP processing essentially ruling out the possibility of off-target antibody effects in our model systems. Importantly, 2B3 antibody characterization ( Supplementary Fig. S4 ) indicated no detectable binding to endogenous murine APP, Aβ and CTF species, further confirming the specificity of this antibody. Previous reports, in combination with these data presented here, altogether supported our hypothesis that sAPP-α directly mediates suppression of Aβ generation. Based on our findings that sAPP-α binds and interferes with BACE1-mediated APP processing, suppression of sAPP-α likely results in BACE1 disinhibition. These results implicate decreased sAPP-α as a potential pathologic determinant in AD pathogenesis. These properties of sAPP-α appeared to depend in part on the secondary and tertiary structure of sAPP-α given that heat-inactivated sAPP-α lost its ability to suppress Aβ production or interfere with BACE1/APP interaction ( Supplementary Fig. S3 ). Additionally, the possibility that sAPP-α is binding to and interfering with full-length APP [32] , [33] , [34] or β-CTF rather than BACE1 exists, but in our model systems is unlikely, given negative IP/IB data suggesting that sAPP-α did not interact well with full-length APP or β-CTF ( Supplementary Fig. S3c and S3d ). Perhaps most importantly, in PSAPP mouse model (human mutant APPK595N/M596 L [APP swe ] and PS1 ΔE9 overexpressing mice), sAPP-α overexpression led to reduced levels of detergent soluble and insoluble Aβ ( Fig. 6a ), decreased β-CTF production ( Fig. 6b ) and ameliorated brain β-amyloid plaques ( Fig. 5 ), as well as reduced BACE1/APP binding indicating that in vivo sAPP-α can regulate APP processing via interactions with BACE1 ( Fig. 6c and d ). Finally, i.c.v. administration of an anti-C-terminal sAPP-α-specific 2B3 antibody in PSAPP mice resulted in exacerbation of amyloidogenic APP processing compared with i.c.v. injection using isotype-matched IgG 2b control antibody ( Fig. 7 ). The results of the present study implicated that inadequate sAPP-α levels are likely sufficient to polarize APP processing towards the amyloidogenic, Aβ producing route due to dishinhibition of BACE1. β-secretase cleavage is considered to be the rate-limiting step in the generation of Aβ. While direct inhibition of BACE shows promise for the treatment of AD, other BACE substrates, including the proteins involved in control of myelination [49] , [50] , [51] , [52] , [53] , [54] , [55] , could be affected by non-selectively inhibiting BACE1 activity. In sum, we suggested a novel mechanism of APP autoregulation via sAPP-α, which appears to attenuate Aβ formation under the physiological condition. If this endogenous sAPP-α-mediated BACE1 inhibition is disturbed, pathologic Aβ generation may ensue. We have confirmed this mechanism through multiple modalities both in vitro and in three mouse models whereby there is a physical interaction between sAPP-α and BACE1; an event that in AD patients may precede the generation of toxic Aβ species. Development of selective BACE modulators, interventions to restore sAPP-α's BACE modulation functions, or sAPP-α mimetics could hold therapeutic value as AD prophylactics or therapeutics. Reagents and antibodies Human HEK293-expressed human sAPP-α (hsAPP-α) was generated and purified as previously described [15] , [35] , [40] , [41] . Briefly, hsAPP-α was purified through successive FPLC steps with heparin–sepharose and TSK-gel DEAE-SPW columns. The identity of hsAPP-α was confirmed by IB, and apparent homogeneity was evidenced by silver staining after SDS–PAGE gel electrophoresis and subsequently tested negative for the presence of endotoxins. Heat inactivation was conducted at 100 °C for 5 min and confirmation of the apparent homogeneity of heat-inactivated hsAPP-α was demonstrated by Coomassie Blue visualization after gel electrophoresis and IB for sAPP-α ( Supplementary Fig. S4a ). For cell treatments and i.c.v. injections, sterile, azide-free and low endotoxin antibodies were used, including anti-C-terminal human sAPP-α-specific antibody (2B3, 100 μg ml −1 ; IBL, Minneapolis, MN, USA), Aβ 1−17 antibody (6E10, 1 mg ml −1 ; Covance, Emeryville, CA, USA) and isotype-matched control IgG antibodies (1 mg ml −1 ; BioLegend, San Diego, CA, USA). This sAPP-α-specific 2B3 antibody was further characterized in our in vitro and in vivo systems indicating that this antibody neither recognizes Aβ nor full-length APP ( Supplementary Fig. S4b–f ). Other antibodies include: mouse monoclonal BACE1 antibody (1 mg ml −1 ; Millipore, Billerica, MA, USA); rabbit polyclonal BACE1 antibody and APP C-terminal antibody (500 μg ml −1 ; EMD Biosciences, La Jolla, CA, USA); APP N-terminus antibody (100 μg ml −1 , Millopore); Aβ 17−24 antibody (1 mg ml −1 ; 4G8, Covance) and Aβ 1−12 antibody (BAM10, 500 μg ml −1 ; Sigma-Aldrich, St. Louis, MO, USA); β-actin antibody (100 μg ml −1 ; Sigma-Aldrich); rabbit anti-APP C-terminus polyclonal antibody (500 μg ml −1 ; pAb369) generously provided by Dr Sam Gandy; rabbit anti-APP C-terminus polyclonal antibody (pAb751/770, 100 μg ml −1 ; Calbiochem); rabbit polyclonal oligomer/conformational (OC) antibody (500 μg ml −1 ) was provided by Dr Suhail Rasool and Dr Charles G. Glabe at the University of California. Cell culture CHO cells engineered to express wild-type human APP (CHO/APP wt ), or Swedish mutant human APP (APP swe ), and wild-type human PS1 (CHO/APP swe /PS1 wt ) were kindly provided by Dr. Stefanie Hahn and Dr. Sascha Weggen, (University of Heinrich Heine, Düsseldorf, Germany). SH-SY5Y cells expressing APP swe and wild-type human PS1 (SH/APP swe /PS1 wt ) was a gift from Dr Wataru Araki (National Institute of Neuroscience, Tokyo, Japan). These cells were cultured as described previously [56] , [57] with minor modifications. Mice Transgenic mice overexpressing hsAPP-α were generated at H. Lee Moffitt Cancer Center (Tampa, FL, USA) by pronuclear injection utilizing standard methods. Briefly, the pcDNA3.1 plasmid containing hsAPP-α based on the predicted α-secretase cleavage of the 695 amino-acid isoform of APP (hsAPP-α695) predominant in human CNS was obtained (Dr. Steven Barger, University of Arkansas). To facilitate CNS expression of hsAPP-α, hsAPP-α695 was cut from the pcDNA3.1 plasmid and cloned into the prion promoter-driven MoPrP.Xho vector [58] , [59] . The resulting construct was analysed for proper insertion and alignment by PCR. After this confirmation, the final construct was linearized to remove the plasmid backbone before injection into oocytes. Next, sAPP-α transgenic mice were generated by injection of gel-purified DNA into C57BL/6J×C3H/HeJ F2 embryos. Several lines of transgenic mice were generated. The line with the highest level of sAPP-α protein expression by IB was selected and maintained by heterozygous backcrossing on the C57BL6/J mouse strain for at least 12 generations before experimental use. Genotyping of TgsAPP-α mice was conducted by quantitative real-time PCR using the following sequences of primers: hsAPP-α forward, 5′-GCCTGGACGATCTCCAGC-3′; hsAPP-α reverse, 5′-TGGCCCGGTGTTAGCACTGGC-3′; β-actin forward, 5′-AGCTTGCTGTATTCCCCTCCATCGTG-3′; and β-actin reverse, 5′-AATTCGGATGGCTACGTACATGGCTG-3′. Human mutant APPK 595N/M596L (APP swe ) and PS1 ΔE9 overexpressing (PSAPP) mice were purchased (The Jackson Laboratory, Bar Harbor, ME, USA). Triple transgenic PSAPP/TgsAPP-α mice and littermates were generated and genotyped as described above and previously [59] . Animals were housed and maintained at the University of South Florida (USF), and all experiments were in compliance with protocols approved by the USF Institutional Animal Care and Use Committee. Tissue preparation Mice were euthanized with isoflurane anaesthesia and then transcardially perfused with ice-cold phosphate-buffered saline (PBS). Brains were rapidly isolated and one hemisphere was frozen immediately in liquid nitrogen and stored at −80 °C. For molecular analysis, brain hemispheres were sonicated in RIPA buffer (Cell Signaling Technology, Danvers, MA, USA) and centrifuged at 14,000 r.p.m. for 1 h at 4 °C. Supernatant was transferred to a new tube for soluble Aβ analysis and pellet was used for insoluble Aβ extraction as described previously [60] . The other hemisphere was placed in 4% paraformaldehyde in PBS for cryostat sectioning. The 25-μm free-floating coronal sections were collected and stored in PBS with 100 mM sodium azide in 24-well plates at 4 °C. IB and IP Cells were washed with ice-cold PBS three times, then lysed with cell lysis buffer (Cell Signaling Technology) and kept at −80 °C until use. Aβ species secreted from cells and from brain homogenates were analysed by Aβ immunoblotting (IB) analysis [60] . Briefly, 10% bicine/tris gel containing 8 M urea was used for separation of proteins from brain homogenates or CHO cell supernatants. Proteins were then transferred to 0.2 μm pore-size nitrocellulose membrane (Bio-Rad, Hercules, CA, USA). The membrane was boiled in PBS for 3–5 min before blocking to enhance sensitivity. 6E10 was used for detection of Aβ. 6E10 and BAM10 were used for detection of Aβ. The 4–20% precast polyacrylamide gels (Bio-Rad, Richmond, CA, USA) were used for APP C-terminal antibody, and 16.5% Tris-tricine gels were used for pAb369 and pAb751/770. The 10% Tris-SDS gels were used for all other antibodies detection. Densitometry analysis was done as previously described using a FluorS Multiimager with Quantity One™ software [60] . Immunoprecitipation (IP) was performed by first incubating conditioned media or brain homogenates with appropriate antibodies and Protein-G Sepharose beads (1:10, Sigma-Aldrich) overnight with gentle rocking at 4 °C. Following three washes with 1× cell lysis buffer, samples were subjected to IB as described above. ELISA Aβ 40, 42 species from cell systems and brain homogenates were detected by the Aβ 40, 42 ELISA kits (Invitrogen, Carlsbad, CA, USA). The manufacturer's instructions were strictly followed. In addition, for the 6E10 immunodepletion experiments, we have established an alternative procedure to measure Aβ 40, 42 levels in the cultured media. Briefly, rabbit polyclonal anti-Aβ 32–40 antibody (Abcam, Cambridge, MA, USA; 5 μg ml −1 in PBS) was used for coating the 96-well plate at 4 C with overnight incubation. Following three washes (PBS with 0.05% Tween-20), blocking buffer (1% bovine serum albumin in PBS) was applied for 2 h at ambient temperature. Next, the plate was washed four times and samples (cell cultured media) were applied to the plate for overnight incubation at 4 °C. After washing, 6E10 (2 μg ml −1 ) was added to the plate for 2 h incubation at ambient temperature to bind Aβ. Finally, following four washes, HRP-conjugated goat anti-mouse IgG (0.5 μg ml −1 ; Cell Signaling Technology) was used for detection and developed with TMB substrate–chromogen (Dako, Carpinteria, CA, USA), then stopped with 2 N sulphuric acid and read spectrophotometrically at 450 nm. The Aβ 40, 42 levels are represented as relative fold OD reading mean (±s.d.) over control. Immunohistochemistry Brain sections from PSAPP and PSAPP/sAPP-α mice were stained with 4G8 or OC antibody. Aβ burden was determined by quantitative image analysis as described previously [60] . Briefly, images of five sections (150 μm apart) through each anatomic region of interest were captured and a threshold optical density was obtained that discriminated staining from background. Manual editing of each field was used to eliminate artifacts. Data are reported as percentage of immunolabelled area captured (positive pixels divided by total pixels captured). This was performed by a single examiner (T.M.) blinded to sample identities. I.c.v. injection of sAPP-α targeting antibodies At 8 months of age, three female mice per group were anesthetized using isoflurane (chamber induction at 4–5% isoflurane, intubation and maintenance at 1–2%). After-reflexes were checked to ensure that mice were unconscious, they were positioned on a stereotaxic frame (Stoelting Lab Standard™, Wood Dale, IL) with ear bars positioned and jaws fixed to a biting plate. The axis coordinates were taken from a mouse brain atlas, and a 5-mm sterile plastic guide cannula (Plastic One, Roanoke, VA, USA) was implanted into the left lateral ventricle delimited from the stereotaxic coordinates (coordinates relative to bregma: −0.6 mm anterior/posterior, +1.2 mm medial/lateral and −3.0 mm dorsal/ventral) using the stereotaxic device (Stoelting Lab Standard) and an attached probe holder. Antibodies targeting regions of sAPP-α characterized to contain a unique BACE1 inhibition sequence [44] were i.c.v. injected with anti-C-terminal sAPP-α-specific antibody (2B3), anti-Aβ 1−17 antibody (6E10) or isotype-matched IgG control antibodies (5 μg per mouse administered at the rate of 1 μl min −1 using a Hamilton syringe modified with a solder stop to prevent over-insertion of the needle). The wounds were closed with 1–2 staples and mice were all observed until anaesthesia had cleared. At 48 h after the i.c.v. injections, animals were killed with isoflurane and brain tissues collected. All dissected brain tissues were rapidly frozen for analysis. Statistical analysis All data were normally distributed; therefore, in instances of single mean comparisons, Levene's test for equality of variances followed by t -test for independent samples was used to assess significance. In instances of multiple mean comparisons, analysis of variance was used, followed by post-hoc comparison using Bonferonni's method. Alpha levels were set at 0.05 for all analyses. The statistical package for the social sciences release 10.0.5 (SPSS, Chicago, IL, USA) was used for all data analysis. How to cite this article: Obregon, D. et al . Soluble amyloid precursor protein-α modulates β-secretase activity and amyloid-β generation. Nat. Commun. 3:777 doi: 10.1038/ncomms1781 (2012).